Divergent rhodium-catalyzed electrochemical vinylic C–H annulation of acrylamides with alkynes α-Pyridones and α-pyrones are ubiquitous structural motifs found in natural products and biologically active small molecules. Here, we report an Rh-catalyzed electrochemical vinylic C–H annulation of acrylamides with alkynes, affording cyclic products in good to excellent yield. Divergent syntheses of α-pyridones and cyclic imidates are accomplished by employing N- phenyl acrylamides and N- tosyl acrylamides as substrates, respectively. Additionally, excellent regioselectivities are achieved when using unsymmetrical alkynes. This electrochemical process is environmentally benign compared to traditional transition metal-catalyzed C–H annulations because it avoids the use of stoichiometric metal oxidants. DFT calculations elucidated the reaction mechanism and origins of substituent-controlled chemoselectivity. The sequential C–H activation and alkyne insertion under rhodium catalysis leads to the seven-membered ring vinyl-rhodium intermediate. This intermediate undergoes either the classic neutral concerted reductive elimination to produce α-pyridones, or the ionic stepwise pathway to produce cyclic imidates. α-Pyridones and α-pyrones are ubiquitous structural motifs found in natural products and biologically active small molecules [1] , [2] , [3] . Transition metal-catalyzed vinylic C–H annulation of acrylic amides or acrylic acids with alkynes has recently emerged as one of the most powerful tools for their synthesis [4] , [5] , [6] , [7] , [8] , [9] , [10] , [11] , [12] , [13] , [14] , [15] . In 2009, Miura and co-workers described an early example of Rh-catalyzed oxidative coupling of substituted acrylic acids with alkynes using Ag 2 CO 3 as the oxidant, affording α-pyrones [16] . Subsequently, the groups of Li and Rovis reported Rh-catalyzed vinylic C–H annulation of acrylamides with alkynes to afford α-pyridones under elevated temperature using stoichiometric transition metal oxidants (Fig. 1a , left side) [17] , [18] . Inspired by these seminal works, various transition metal-catalyzed vinylic C–H annulation reactions with alkynes have been developed to prepare α-pyridones or α-pyrones, including ones catalyzed by Rh [19] , [20] , [21] , [22] , [23] , [24] , Ru [25] , [26] , [27] , [28] , [29] , Co [30] , [31] , [32] , [33] , Pd [34] , [35] , [36] , and Fe [37] , [38] catalysts. Despite these advances, important challenges remain, including: (1) typically high reaction temperatures (100–120 °C); (2) stoichiometric transition metal oxidants such as Cu(OAc) 2 or AgOAc are generally required to regenerate catalysts; (3) a highly selective divergent synthesis of α-pyridones and cyclic imidates (Fig. 1a , right side) from acrylamides is still lacking [17] . Fig. 1: Rh-catalyzed vinylic C–H annulation of acrylamides with alkynes to afford α-pyridone and cyclic imidate. a Rh-catalyzed vinylic C–H annulation under elevated temperature with stoichiometric transition metal oxidants. b Rh-catalyzed electrochemical vinylic C–H annulation of acrylamides with alkynes. Full size image Electrochemical organic synthesis has received tremendous attention because electric current offers an environmentally benign alternative to conventional methods for oxidation and reduction of organic compounds, such as those involving chemical oxidants and reductants [39] , [40] , [41] , [42] , [43] , [44] , [45] , [46] , [47] , [48] , [49] , [50] , [51] , [52] , [53] , [54] , [55] , [56] , [57] , [58] , [59] , [60] . Transition metal-catalyzed electrochemical arene C–H annulation with alkynes has been developed using catalysts including Co [61] , [62] , [63] , [64] , Ru [65] , [66] , [67] , [68] , [69] , [70] , [71] , Rh [72] , [73] , [74] , and Cu [75] . In contrast, electrochemical vinylic C–H annulation with alkynes is less studied. Recently, we reported an Ir-catalyzed electrochemical vinylic C–H annulation reaction of acrylic acids with internal alkynes, affording α-pyrones in good yields, but terminal alkynes are not tolerated [76] . Subsequently, Ackermann and co-workers demonstrated Ru-catalyzed electrochemical vinylic C–H annulation of acrylamides with symmetric internal alkynes at elevated temperature (140 °C) [77] . Herein, we report an Rh(III)-catalyzed electrochemical vinylic C–H annulation of acrylamides with alkynes in an undivided cell under mild reaction conditions. Importantly, divergent syntheses of α-pyridones and cyclic imidates are achieved by varying the N- substituent of the acrylamides. Furthermore, terminal alkynes are well tolerated in this Rh-catalyzed electrochemical vinylic C–H annulation (Fig. 1b ). We also probed the reaction mechanism by carrying out cyclic voltammetric analysis and kinetic isotopic experiments. Density functional theory (DFT) calculations elucidated origins of substituent-controlled chemoselectivity. The sequential C–H activation and alkyne insertion under rhodium catalysis leads to the seven-membered ring vinyl-rhodium intermediate. This intermediate undergoes either the classic neutral concerted reductive elimination to produce pyridones, or the ionic stepwise pathway to produce cyclic imidates. The electronic nature of the N- substituent has exactly the reversal effect on the rates of neutral concerted and ionic stepwise reductive elimination pathways, which switches the chemoselectivity. 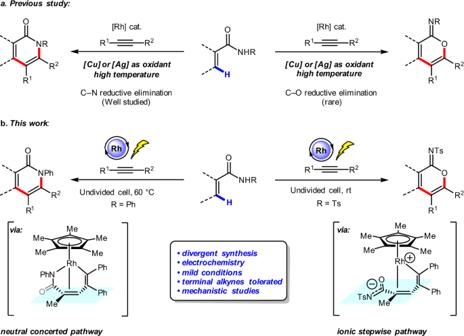Fig. 1: Rh-catalyzed vinylic C–H annulation of acrylamides with alkynes to afford α-pyridone and cyclic imidate. aRh-catalyzed vinylic C–H annulation under elevated temperature with stoichiometric transition metal oxidants.bRh-catalyzed electrochemical vinylic C–H annulation of acrylamides with alkynes. Optimization studies Initially, we probed various reaction conditions using 2-methylacrylamide ( 1a ) and diphenylacetylene ( 2a ) as reaction partners in an undivided cell (Table 1 and Supplementary Tables 1 – 7 ). To our delight, using (Cp*RhCl 2 ) 2 as the precatalyst, n -Bu 4 NOAc as the electrolyte, and MeOH as the solvent in an undivided cell with two platinum electrodes under constant-current electrolysis at 1.5 mA for seven hours at 60 °C, cyclic imidate 3a can be obtained in 91% isolated yield (Table 1 , entry 1). Acetonitrile as solvent affords a similar yield, while yield diminishes significantly when other solvents are used (entries 2−5). Other electrolytes such as NaOAc and NaOPiv result in slightly lower yields (entries 6 and 7). Control experiments show that no significant amount of annulation product is produced in the absence of the catalyst or electric current (entries 8 and 9). To our delight, 92% isolated yield is obtained when the reaction is carried out with IKA ElectraSyn 2.0 at room temperature (entry 10) [78] . Furthermore, changing the electrode material caused a small decrease in yield (entries 11 and 12). Interestingly, switching to the synthesis of α-pyridones instead of cyclic imidates can be achieved by simply changing the N- substitution of acrylamides (entries 13–15). α-Pyridone 4b can be obtained in 95% isolated yield when N- phenyl acrylamide 1b is used (entry 13). Other N- aryl groups afford lower yields with good selectivity of α-pyridones versus cyclic imidates (entries 14 and 15). Table 1 Annulation optimization with acrylamide 1a and diphenylacetylene a . Full size table Scope of cyclic imidates With the optimized reaction conditions in hand, we investigated the generality of this electrochemical C–H annulation. As shown in Fig. 2a , various acrylamides substituted with alkyl, ester, ether, aryl, fluoro, chloro, and bromo groups are well tolerated, affording the corresponding cyclic imidates in good to excellent yields ( 3a , 6a – 6r ). Unfortunately, β-substituted substrate like cinnamide-derived acrylamides give lower yields, which could be due to the steric effects (see Supplementary information for more details). A variety of alkynes react well, including diarylacetylenes ( 7a – 7l ) and dialkylacetylenes ( 7m – 7o ). With unsymmetrical alkynes, regioselectivity is governed by arene electronics. For example, moderate regioselectivity is achieved with n -butyl phenyl acetylene ( 7p ). Fig. 2: Scope of cyclic imidates and synthetic application. a Substrate scope synthesis of cyclic imidates with IKA Electrasyn 2.0. a Isolated yields are reported. Reaction conditions: 1a or 5 (0.3 mmol), 2 (0.2 mmol), (Cp*RhCl 2 ) 2 (4 mol%), n -Bu 4 NOAc (3.0 equiv. ), and MeOH (6 mL) in an undivided cell with two platinum electrodes (each 3.0 × 0.8 cm 2 ), room temperature, 1.5 mA, 7–12 h. b 5 (0.15 mmol), 2 (0.3 mmol). c The reaction was carried out at 60 °C. b Gram-scale experiment and synthetic application. Full size image In contrast, excellent regioselectivities are obtained when electron-deficient arylacetylenes are employed ( 7q and 7r ). In addition, excellent regioselectivities and yields are accomplished using terminal alkynes, with the alkyl or aryl groups oriented proximal to the oxygen heteroatom in the product ( 7s – 7x ). (As a reminder, terminal alkynes are not tolerated in the aforementioned Ir-catalyzed electrochemical C–H annulation [76] .) Furthermore, the structures of 3a , 6c , 6o , 7r , and 7s were unambiguously verified by X-ray analysis. Finally, we demonstrated the preparative utility of this Rh-catalyzed electrochemical C–H annulation reaction by running a reaction containing 6.0 mmol of substrate 1a and 4.0 mmol of substrate 2a to afford cyclic imidate 3a in 86% yield, which can be further converted into α-pyrone 3aa (Fig. 2b ). Scope of α-pyridones We also examined the reactivity of a series of substituted acrylamides and alkynes for the synthesis of α-pyridones (Fig. 3 ). Acrylamides bearing a variety of functional groups such as alkyl, ester, ether, and aryl are well tolerated under the standard reaction conditions, affording α-pyridones in moderate to good yields ( 4b , 9a − 9l ). Fig. 3: Scope of α-pyridones. Isolated yields are reported. Reaction conditions: 1b or 8 (0.3 mmol), 2 (0.2 mmol), (Cp*RhCl 2 ) 2 (4 mol%), n -Bu 4 NOAc (3.0 equiv.) and MeOH (3 mL), in an undivided cell with two platinum electrodes (each 1.0 × 1.0 cm 2 ), 60 °C, 1.5 mA, 7–12 h. Full size image A series of experiments were carried out to elucidate the mechanism of this electrochemical C–H annulation reaction. First, acrylamide 1a was subjected to the electrochemical C–H annulation reaction conditions in CH 3 OD in the absence of an alkyne. Significant H/D exchange was observed, indicating that the putative C–H activation step is reversible (Fig. 4a ). A kinetic isotope effect (KIE) value was determined by comparing parallel experiments using acrylamide 5e and corresponding deuterated substrate 5e- d 4 (Fig. 4b ). A KIE value of 1.4 was observed (see Supplementary information for details). In addition, we executed the stoichiometric reaction of acrylamides, diphenylacetylene 2a , and (Cp*RhCl 2 ) 2 in the absence of electric current. To our delight, the rhodium sandwich complexes 10 and 11 were obtained in good yield, with the corresponding cyclic imidate as a neutral η4 ligand. Their structures were unambiguously confirmed by X-ray analysis (Fig. 5a ). Upon anodic oxidation, the product 3a is released from 10 , and is a coordinatively saturated, 18-electron complex (Fig. 5b ). Additionally, 3a is obtained in good yield when a catalytic amount of 10 is employed, which suggests that 10 is a competent intermediate and catalyst in this electrochemical C–H annulation (Fig. 5c ). Fig. 4: H/D exchange experiment and kinetic isotopic effect experiments. a H/D exchange experiment. b Kinetic isotopic effect experiments. Full size image Fig. 5: Stoichiometric reaction. a Stoichiometric reactions in the absence of electric current. b Anodic oxidation of complex 10 . c Catalytic reaction with complex 10 . Full size image Complex 10 in 0.1 M solution of n -Bu 4 NPF 6 in MeCN exhibits the first oxidation peak at 0.70 V versus saturated calomei electrode (curve d, Fig. 6 ), which is significantly lower than the oxidation potentials for the oxidation of other components in the reaction system (Fig. 6 ). This supports the hypothesis that the role of anodic oxidation is to oxidize a diene-Rh(I) complex to an active Rh(III) species with concomitant release of the product. Fig. 6: Cyclic voltametric study. Cyclic voltammograms recorded on a Pt electrode (area = 0.03 cm 2 ) with a scan rate of 100 mV s − 1 : a MeCN containing 0.1 M n -Bu 4 NPF 6 ; b MeCN containing 0.1 M n -Bu 4 NPF 6 , after addition of 4 mM 3a ; c MeCN containing 0.1 M n -Bu 4 NPF 6 , after addition of 4 mM 1a ; d MeCN containing 0.1 M n -Bu 4 NPF 6 , after addition of 4 mM 10 ; e MeCN containing 0.1 M n -Bu 4 NPF 6 , after addition of 4 mM complex (Cp*RhCl 2 ) 2 ; f MeCN containing 0.1 M n -Bu 4 NPF 6 , after addition of 4 mM 2a . Full size image We next explored the reaction mechanism and the origins of substrate-controlled chemoselectivity through DFT calculations (see Supplementary information and Supplementary Data 1 for more details). From the active catalyst Cp*Rh(OAc) 2 , sequential vinyl C–H activation of N- tosyl acrylamide 1a and diphenylacetylene insertion generate the seven-membered ring vinyl–rhodium intermediate int1 (Supplementary Fig. 14 and Fig. 7 ) [79] , [80] . Int1 can undergo competing reductive eliminations to form either the α-pyridone product or cyclic imidate (Fig. 7 ). The classic neutral concerted reductive elimination (red pathway) occurs through the three-membered ring transition state TS2 , generating the α-pyridone product-coordinated complex int3 . This neutral concerted reductive elimination requires an insurmountable barrier of 31.6 kcal/mol, which is unfeasible under the experimental conditions. Alternatively, we found that the ionic stepwise pathway (black pathway) can be operative and produce the cyclic imidate product. This ionic stepwise pathway, discovered by Hong group [81] in similar transformation under ruthenium catalysis, initiates through a heterolytic cleavage of the rhodium-nitrogen bond via TS5 with the assistant of methanol to generate the zwitterionic intermediate int6 . From int6 , methanol dissociates to generate int7 , subsequent facile C–O bond formation through TS8 (IRC conformation of TS8 is included in the Supplementary information ) produces int9 . The zwitterionic species int7 also has the possibility for rhodium-oxygen bond formation via TS10 (labeled in purple), but requiring a higher barrier as compared to the C–O bond formation. 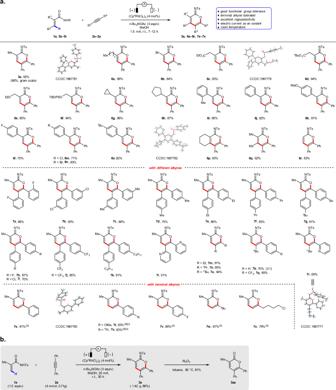Fig. 2: Scope of cyclic imidates and synthetic application. aSubstrate scope synthesis of cyclic imidates with IKA Electrasyn 2.0.aIsolated yields are reported. Reaction conditions:1aor5(0.3 mmol),2(0.2 mmol), (Cp*RhCl2)2(4 mol%),n-Bu4NOAc (3.0 equiv.), and MeOH (6 mL) in an undivided cell with two platinum electrodes (each 3.0 × 0.8 cm2), room temperature, 1.5 mA, 7–12 h.b5(0.15 mmol),2(0.3 mmol).cThe reaction was carried out at 60 °C.bGram-scale experiment and synthetic application. Comparing the free energy barriers of the two competing pathways, the ionic stepwise reductive elimination is more favorable by 7.7 kcal/mol ( TS2 vs. TS5 ), which is consistent with the experimental chemoselectivity favoring cyclic imidate when N -tosyl acrylamide is employed. Fig. 7: DFT calculations with 1a substrate. DFT-computed free energy changes of competing reductive elimination pathways from seven-membered ring vinyl-rhodium intermediate when N -tosyl acrylamide 1a was employed as substrate. Full size image The DFT-computed free energy changes of the same competing reductive elimination pathways for the N -phenyl acrylamide 1b substrate is shown in Fig. 8 . From N -phenyl acrylamide 1b , the sequential vinyl C–H activation and diphenylacetylene insertion generate the seven-membered ring vinyl-rhodium intermediate int12 (Supplementary Fig. 15 ). This intermediate can undergo the classic neutral concerted reductive elimination pathway via TS13 (red pathway), with a barrier of 21.9 kcal/mol. The alternative ionic stepwise pathway through TS16 (IRC conformation of TS16 is included in the Supplementary information ) is significantly less favorable, due to the unstable zwitterionic species int18 . Comparing to the tosyl substituent, the phenyl substituent significantly lowers the barrier of neutral concerted pathway while increases the barrier of ionic stepwise pathway, which results in the reversal chemoselectivity. For the ionic stepwise pathway, the electron-withdrawing tosyl substituent weakens the rhodium-nitrogen bond of int1 , which favors its heterolytic cleavage and the generation of the zwitterionic intermediate int7 (Fig. 7 ). The same process is endergonic by 27.3 kcal/mol for the N -phenyl substituted case ( int12 to int18 , Fig. 8 ). This electronic effect is further supported by the computed rhodium-nitrogen bond dissociation energies and additional Hammett analysis of the N -substitution (Supplementary Fig. 19 ). For the neutral concerted pathway, our distortion/interaction analysis revealed the distortion-controlled origins of the substituent effect (Supplementary Fig. 18 ). The phenyl substituent induces geometric change of the seven-membered rhodacycle in int12 , leading to the predistortion towards the neutral concerted reductive elimination transition state TS13 . This predistortion is reflected in the highlighted distance of the forming C–N bond in the seven-membered ring intermediates (2.71 Å in int12 , Fig. 8 ; 2.84 Å in int1 , Fig. 7 ). These insights provide a mechanistic basis for rational reaction designs in related transformations. Fig. 8: DFT calculations with 1b substrate. DFT-computed free energy changes of competing reductive elimination pathways from seven-membered ring vinyl-rhodium intermediate int10 when N -phenyl acrylamide 1b was employed as substrate. Full size image Based on our mechanistic studies, we propose a plausible catalytic cycle as shown in Fig. 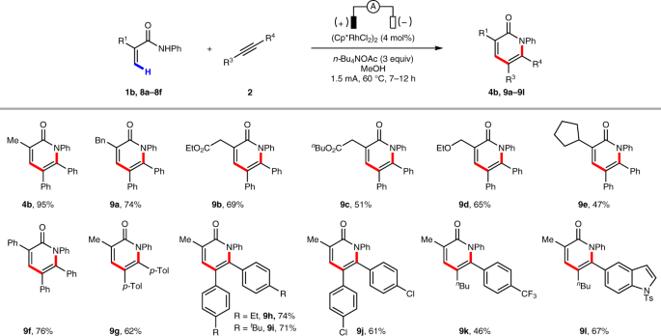Fig. 3: Scope of α-pyridones. Isolated yields are reported. Reaction conditions:1bor8(0.3 mmol),2(0.2 mmol), (Cp*RhCl2)2(4 mol%),n-Bu4NOAc (3.0 equiv.) and MeOH (3 mL), in an undivided cell with two platinum electrodes (each 1.0 × 1.0 cm2), 60 °C, 1.5 mA, 7–12 h. 9 . Initially, C–H activation takes place to afford a cyclometallated Rh(III) intermediate B , following ligand exchange to deliver complex C . Next, migratory alkyne insertion results in the seven-membered rhodium complex D [82] , [83] , which undergoes ionic stepwise or neutral concerted reductive elimination to give Rh(I) complex 10 or E . Intermediate 10 or E is a coordinately saturated, 18-electron complex. Upon anodic oxidation, the product is released from 10 or E , and complex A is regenerated. Fig. 9: Plausible catalytic cycle. The catalytic cycle starts from C–H activation, and then alkyne insertion leads to the seven-membered ring vinyl-rhodium intermediate D . Subsequently intermediate D undergoes either the classic neutral concerted reductive elimination to produce intermediate E , or the ionic stepwise pathway to produce complex 10 . Finally, product formation under anodic oxidation, and complex A is regenerated. Full size image In summary, we have developed an electrochemical method for the Rh(III)-catalyzed vinylic C–H annulation of acrylamides with alkynes. 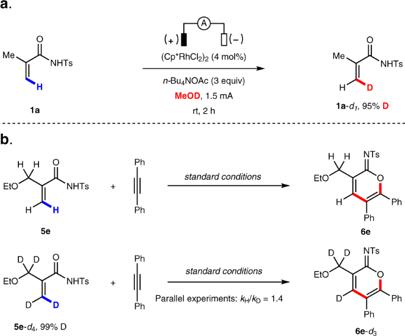Fig. 4: H/D exchange experiment and kinetic isotopic effect experiments. aH/D exchange experiment.bKinetic isotopic effect experiments. Owing to the robustness of this electrochemical C–H annulation, the reaction can be operated with IKA ElectraSyn 2.0 at room temperature, affording cyclic imidates with good to excellent yields. Additionally, divergent syntheses of a-pyridones and cyclic imidates are realized by simply switching the N -substitution of acrylamides. Furthermore, excellent regioselectivities are achieved with unsymmetrical alkynes, including terminal alkynes. Mechanistic and DFT studies combined to provide a rationale for the chemoselectivity switch and a basis for future reaction design in related transformations. General procedure for the electrolysis The electrocatalysis was carried out in an IKA ElectraSyn 2.0 equipped with two platinum electrodes (each 0.8 × 3.0 cm 2 ). Acrylic amide (0.3 mmol, 1.5 equiv. ), alkyne (0.2 mmol, 1.0 equiv. 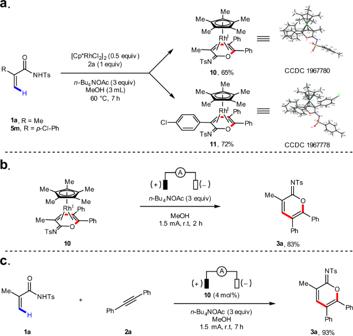Fig. 5: Stoichiometric reaction. aStoichiometric reactions in the absence of electric current.bAnodic oxidation of complex10.cCatalytic reaction with complex10. 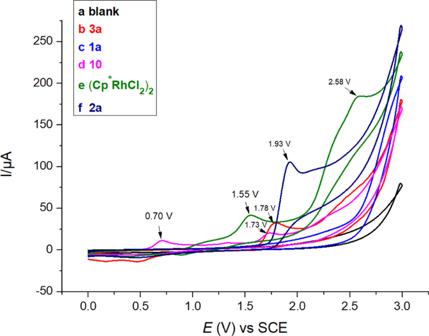Fig. 6: Cyclic voltametric study. Cyclic voltammograms recorded on a Pt electrode (area = 0.03 cm2) with a scan rate of 100 mV s− 1:aMeCN containing 0.1 Mn-Bu4NPF6;bMeCN containing 0.1 Mn-Bu4NPF6, after addition of 4 mM3a;cMeCN containing 0.1 Mn-Bu4NPF6, after addition of 4 mM1a;dMeCN containing 0.1 Mn-Bu4NPF6, after addition of 4 mM10;eMeCN containing 0.1 Mn-Bu4NPF6, after addition of 4 mM complex (Cp*RhCl2)2;fMeCN containing 0.1 Mn-Bu4NPF6, after addition of 4 mM2a. ), n -Bu 4 NOAc (0.6 mmol, 3.0 equiv.) 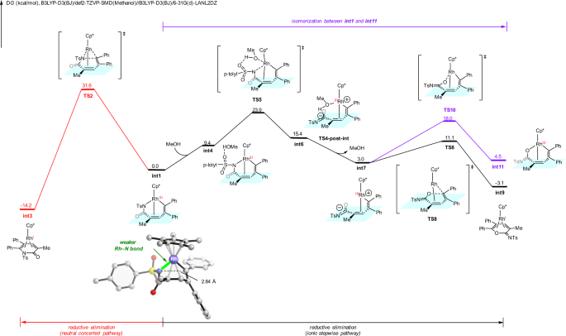Fig. 7: DFT calculations with 1a substrate. DFT-computed free energy changes of competing reductive elimination pathways from seven-membered ring vinyl-rhodium intermediate whenN-tosyl acrylamide1awas employed as substrate. 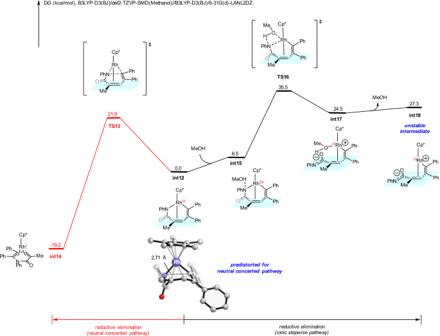Fig. 8: DFT calculations with 1b substrate. DFT-computed free energy changes of competing reductive elimination pathways from seven-membered ring vinyl-rhodium intermediateint10whenN-phenyl acrylamide1bwas employed as substrate. 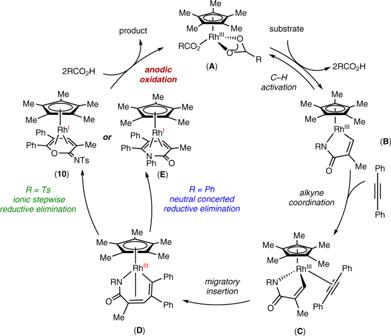Fig. 9: Plausible catalytic cycle. The catalytic cycle starts from C–H activation, and then alkyne insertion leads to the seven-membered ring vinyl-rhodium intermediateD. Subsequently intermediateDundergoes either the classic neutral concerted reductive elimination to produce intermediateE, or the ionic stepwise pathway to produce complex10. Finally, product formation under anodic oxidation, and complexAis regenerated. and (Cp*RhCl 2 ) 2 (4.0 mol%, 99 wt%) were dissolved in MeOH (6.0 mL). Electrocatalysis was performed at room temperature with a constant current of 1.5 mA maintained for 7–12 h (2.0–3.4 F/mol). After the reaction, the mixture was concentrated in vacuo. The resulting residue was purified by silica gel flash chromatography to give the annulation product. More experimental procedures and photographic guide for electrochemical C–H annulation are provided in the Supplementary information .